Structural basis for ion selectivity revealed by high-resolution crystal structure of Mg2+channel MgtE Magnesium is the most abundant divalent cation in living cells and is crucial to several biological processes. MgtE is a Mg 2+ channel distributed in all domains of life that contributes to the maintenance of cellular Mg 2+ homeostasis. Here we report the high-resolution crystal structures of the transmembrane domain of MgtE, bound to Mg 2+ , Mn 2+ and Ca 2+ . The high-resolution Mg 2+ -bound crystal structure clearly visualized the hydrated Mg 2+ ion within its selectivity filter. Based on those structures and biochemical analyses, we propose a cation selectivity mechanism for MgtE in which the geometry of the hydration shell of the fully hydrated Mg 2+ ion is recognized by the side-chain carboxylate groups in the selectivity filter. This is in contrast to the K + -selective filter of KcsA, which recognizes a dehydrated K + ion. Our results further revealed a cation-binding site on the periplasmic side, which regulate channel opening and prevents conduction of near-cognate cations. The magnesium ion, Mg 2+ , is involved in many cellular functions, such as the formation of RNA and protein structures, genome stability and enzymatic catalysis [1] , [2] , and thus is an essential cation for life. The intracellular homeostasis of the Mg 2+ concentration is important for these functions, and thus is maintained by Mg 2+ transporters and channels that translocate Mg 2+ across biological membranes. The cellular concentrations of other biological cations (that is, Na + , K + and Ca 2+ ) are strictly controlled, and thus the selective transport of Mg 2+ by these transporters and channels is of particular importance. The selective transport mechanism of monovalent cations has been well investigated, based on the crystal structures of Na + and K + channels. The atomic resolution crystal structures of KcsA [3] , [4] and MthK [5] revealed that K + is dehydrated and directly recognized by the protein atoms in the selectivity filter. In contrast, the selective transport mechanism for divalent cations, such as Ca 2+ and Mg 2+ , has remained elusive. The dehydration energies of divalent cations are much higher than those of monovalent cations, and thus their recognition mechanisms are attracting significant interest. The crystal structures of divalent cation channels, including CorA [6] , [7] , [8] , [9] , Orai [10] and Ca 2+ conductive Na + channel [11] , suggested that their selectivity filters consist of multiple acidic residues, with carboxylate groups that recognize the divalent cation. However, the medium-resolution structures of these channels limited the clear understanding of the ion recognition mechanism by the selective filters for divalent cations. MgtE is a Mg 2+ channel widely conserved in archaea, bacteria and eukaryotes [12] . The bacterial MgtE is a high-conductance Mg 2+ -selective channel gated by the cytosolic Mg 2+ concentration and is involved in the cellular homeostasis of Mg 2+ . The vertebrate homologues of MgtE are known as the SLC41 family transporters, and the SLC41A1, SLC41A2 and SLC41A3 members of this family were also shown to mediate Mg 2+ transport across the plasma or organellar membranes [13] , [14] . Several mutations related to Parkinson’s disease exist in the SLC41A1 gene [15] . The crystal structures of Thermus thermophilus MgtE revealed that MgtE forms a homodimer, consisting of the cytosolic region and the transmembrane (TM) domain [16] , [17] . The cytosolic region comprises the N domain, the CBS domain and the plug helix. These domains contain several Mg 2+ -binding sites and were suggested to function as sensors for the cytosolic Mg 2+ concentration. The ion-conducting pore is formed at the homodimeric interface of the TM domain, which may selectively recognize Mg 2+ to allow its conduction across the membrane. The cytosolic side of the pore is sealed by the plug helix, while its periplasmic side is closed by the hydrophobic gate, suggesting that the structures represent a closed form. In the ion-conducting pore, Asp432 is the sole acidic residue that is widely conserved in the MgtE family members, including the vertebrate SLC41 transporters. A strong electron density peak was observed around the Asp432 carboxylate groups, suggesting the binding of Mg 2+ . These observations strongly suggested that the site at the middle of the pore including Asp432 functions as the selectivity filter of MgtE [16] , [17] . However, the detailed mechanism of Mg 2+ recognition by the selectivity filter has remained elusive, because the medium resolution of the crystal structures could not distinguish the water molecules coordinated to Mg 2+ . In this study, we determined the crystal structure of the MgtE TM domain (MgtE-TMD) at 2.2 Å resolution. The high-resolution crystal structure clearly revealed the metal ion and its coordinated water molecules bound to the selectivity filter. To our knowledge, this is the first visualization of the fully hydrated divalent cation recognized by the selectivity filter of ion channels. In combination with biochemical analyses, we proposed the divalent cation selectivity mechanism by MgtE. Crystal structure of MgtE-TMD In the previously determined full-length structure of MgtE, the ion-conducting pore is formed at the dimer interface, which harbours two conserved Asp residues (Asp432 in TM5) in the middle of the TM segment (M1 site, Fig. 1a ). This M1 site is mainly composed of TM2 and TM5, and is expected to function as a Mg 2+ -specific selectivity filter [16] . To obtain high-resolution structural information about the MgtE selectivity filter, we crystallized the TM domain of MgtE (278–450; MgtE-TMD), using the lipidic cubic phase method [18] , [19] . 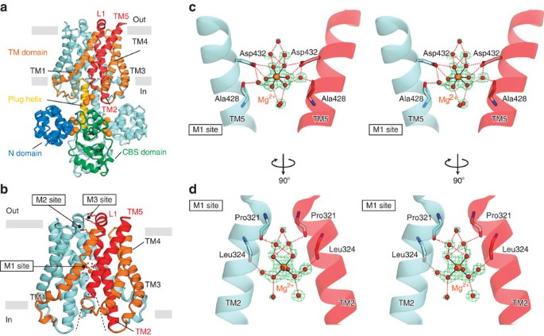Figure 1: High-resolution crystal structure of MgtE-TMD. (a) The full-length MgtE dimer (PDB ID 2ZY9) reported previously16is viewed in the plane of the membrane, highlighting the N domain (blue), CBS domain (green), plug helix (yellow) and pore forming helices, TM2, TM5 and L1 (red), and other helices of TM5 (orange) in one subunit. The other subunit is coloured cyan. (b) The high-resolution structure of the MgtE-TMD dimer bound to Mg2+. The rectangles indicate the divalent cation-binding sites. The overall structure is in the closed conformation. (c,d) Stereo view around TM5 (c) and TM2 (d) of the M1 site, with the 2mFo−DFcelectron density map contoured at 4.0 σ. The coordinate and hydrogen bonds are depicted by solid and dashed lines, respectively. Water molecules and Mg2+ions are represented by red and orange spheres, respectively. We finally determined the crystal structures of MgtE-TMD, bound to Mg 2+ , Mn 2+ and Ca 2+ , at 2.3, 2.2 and 3.2 Å resolutions, respectively ( Table 1 ). The overall structures of MgtE-TMD are essentially the same as the full-length structure determined at 2.94 Å resolution [16] , with a root mean squared deviation of 1.30 Å for all Cα atoms ( Fig. 1a,b ). The hydrophobic gate located just above the M1 site is closed similar to that in the full-length structure. In contrast, the M1 site is accessible from the cytoplasmic side, as MgtE-TMD lacks the plug helix and the cytosolic domain ( Fig. 1b ). Figure 1: High-resolution crystal structure of MgtE-TMD. ( a ) The full-length MgtE dimer (PDB ID 2ZY9) reported previously [16] is viewed in the plane of the membrane, highlighting the N domain (blue), CBS domain (green), plug helix (yellow) and pore forming helices, TM2, TM5 and L1 (red), and other helices of TM5 (orange) in one subunit. The other subunit is coloured cyan. ( b ) The high-resolution structure of the MgtE-TMD dimer bound to Mg 2+ . The rectangles indicate the divalent cation-binding sites. The overall structure is in the closed conformation. ( c , d ) Stereo view around TM5 ( c ) and TM2 ( d ) of the M1 site, with the 2 mF o − DF c electron density map contoured at 4.0 σ. The coordinate and hydrogen bonds are depicted by solid and dashed lines, respectively. Water molecules and Mg 2+ ions are represented by red and orange spheres, respectively. Full size image Table 1 Data collection and refinement statistics. Full size table Structure of the selectivity filter The Mg 2+ -bound structure revealed a strong electron density peak surrounded by six weaker satellite peaks in the M1 site ( Fig. 1c and Supplementary Fig. 1 ). Given that the Mg 2+ ion adopts an octahedral geometry coordinating six water molecules [20] , the present crystal structure indicates that the fully hydrated Mg 2+ ion is bound to the M1 site. 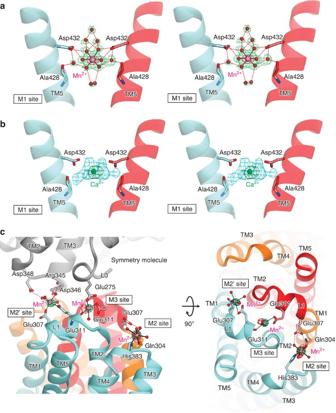Figure 2: Mn2+and Ca2+binding sites in MgtE-TMD. (a) Stereo view of TM5 in the M1 site of the Mn2+-bound structure. The anomalous difference Fourier map derived from the Mn-peak data set contoured at 5.0 σ and the 2mFo−DFcelectron density map contoured at 3.5 σ are shown in magenta and green, respectively. Water molecules and Mn2+ions are represented by red and purple spheres, respectively. (b) Stereo view of TM5 in the M1 site of the Ca2+-bound structure, with the 2mFo−DFcandmFo–DFcelectron density maps contoured at 2.5 σ (green) and 3.0 σ (blue), respectively. Ca2+ions are represented by green spheres. (c) Mn2+binding to the M2, M2′ and M3 sites. Water molecules and Mn2+ions are represented by red and purple spheres, respectively. Amino acid residues involved in binding to Mn2+or hydration water molecules are shown in ball and stick representations. The adjacent MgtE-TMD molecule is coloured grey. The 2mFo−DFcmap (2.5 σ) and anomalous difference Fourier maps (4.5 σ) are shown in green and magenta, respectively. The coordinate and hydrogen bonds are depicted by solid and dashed lines, respectively. The distances between the Mg 2+ ion and the coordinated water molecules are 1.97–2.20 Å ( Table 2 ) and are comparable to the typical Mg-O distance (2.1 Å) in an aqueous environment [20] . This assignment is also consistent with the fact that the crystallization conditions contained 100 mM Mg 2+ . The four carboxylate oxygen atoms of Asp432 hydrogen bond with four of the six water molecules in the first hydration shell, thereby anchoring the fully hydrated Mg 2+ ion to the M1 site ( Fig. 1c ). Besides the first hydration shell, the water molecules in the second hydration shell are also recognized in the M1 site. In addition to the carboxyl oxygen atoms of Asp432, the backbone carbonyl oxygen atoms of Pro321 and Leu324 in TM2, and Ala428 in TM5 are within hydrogen-bonding distance of the water molecules in the second hydration shell ( Fig. 1c,d ). The Gly and Pro residues clustered in the centre of TM2 would confer flexibility to the helix ( Supplementary Fig. 2 ), which might allow the backbone carbonyl groups in the α-helix region to form bifurcated hydrogen bonds with both the water molecules and backbone amide groups. These structural elements involved in the Mg 2+ recognition are also conserved in the human SLC41 transporters ( Supplementary Fig. 2 ), suggesting that they also recognize divalent cations in a similar manner. Table 2 Overview of the M 2+ –O distance and O–M 2+ –O bond angle in the M1 site. Full size table The Mn 2+ ion assumes an octahedral hydration geometry similar to that of Mg 2+ . The structure of the Mn 2+ -bound form revealed that the Mn 2+ ion is also bound to the M1 site in a fully hydrated state, with six water molecules ( Fig. 2a ). In the anomalous difference Fourier map calculated from another data set collected at the peak wavelength for Mn (1.45 Å), we observed a strong peak at the M1 site (11.0 σ, Fig. 2a ), supporting the Mn 2+ binding at this site. Although the manner of Mn 2+ binding to the M1 site is quite similar to that of the Mg 2+ ion, the octahedral geometry of the coordinated water molecules is slightly distorted in this Mn 2+ -bound form ( Table 2 ). The distances between the Mn 2+ ion and the coordinated water molecules are 1.96–2.28 Å. Figure 2: Mn 2+ and Ca 2+ binding sites in MgtE-TMD. ( a ) Stereo view of TM5 in the M1 site of the Mn 2+ -bound structure. The anomalous difference Fourier map derived from the Mn-peak data set contoured at 5.0 σ and the 2 mF o − DF c electron density map contoured at 3.5 σ are shown in magenta and green, respectively. Water molecules and Mn 2+ ions are represented by red and purple spheres, respectively. ( b ) Stereo view of TM5 in the M1 site of the Ca 2+ -bound structure, with the 2 mF o − DF c and mF o – DF c electron density maps contoured at 2.5 σ (green) and 3.0 σ (blue), respectively. Ca 2+ ions are represented by green spheres. ( c ) Mn 2+ binding to the M2, M2′ and M3 sites. Water molecules and Mn 2+ ions are represented by red and purple spheres, respectively. Amino acid residues involved in binding to Mn 2+ or hydration water molecules are shown in ball and stick representations. The adjacent MgtE-TMD molecule is coloured grey. The 2 mF o − DF c map (2.5 σ) and anomalous difference Fourier maps (4.5 σ) are shown in green and magenta, respectively. The coordinate and hydrogen bonds are depicted by solid and dashed lines, respectively. Full size image In the Ca 2+ -bound structure, a strong density peak was observed in the M1 site ( Fig. 2b ), which probably arises from the Ca 2+ ion contained in the crystallization conditions. The distances between the centre of the density peak and the carboxylate oxygen atoms of Asp432 are ~4 Å, suggesting that the Ca 2+ ion is bound to this site in a fully hydrated state, as in the cases of the Mg 2+ and Mn 2+ ions. We observed broad peaks around Ca 2+ in the mF o – DF c density map ( Fig. 2b ); however, we could not model water molecules into these density peaks, because of the medium resolution. The coordination geometry of the Ca 2+ ion is dynamic and exhibits a broad range of coordination numbers, that is, six to eight water molecules, in an aqueous environment [21] , [22] , [23] . This is quite different from those of the Mg 2+ and Mn 2+ ions, which assume rather stable first hydration shells with six water molecules. This difference may result in an unstable interaction of Ca 2+ with the M1 site, and thus explain the lower resolution of the Ca 2+ -bound structure. Overall, these structures suggested that the M1 site specifically recognizes divalent cations that can assume an octahedral geometry, such as Mg 2+ and Mn 2+ . Structure of the periplasmic metal-binding sites In the crystal structure of the Mn 2+ -bound form, we observed three strong peaks around the periplasmic side of MgtE-TMD in the electron density map (M2, M2′ and M3 sites, Fig. 2c ). We also observed strong peaks at the M2 and M3 sites in the anomalous difference Fourier map (4.8 and 4.0 σ, respectively; Supplementary Fig. 3b,e ). These observations suggested that the Mn 2+ ions are bound to these periplasmic sites. The M2 and M2′ sites are located on the surface of the periplasmic side and are related by the twofold non-crystallographic symmetry (NCS) axis between the MgtE-TMD protomers ( Fig. 2c ). The M2 site is not involved in any crystal-packing interactions, while the Mn 2+ ion in the M2′ site forms interactions with an adjacent molecule in the crystalline lattice ( Fig. 2c ). Consequently, the ligand atoms of the M2 site are different from those of the M2′ site. The M2 site consists of the side chains of Gln304 and Glu307 in one protomer and His383 in another protomer ( Supplementary Fig. 3b ). The Mn 2+ ion bound to the M2 site is directly coordinated by the imidazole nitrogen of His383 and the side-chain carbonyl oxygen of Gln304. The Mn 2+ ion is further surrounded by four satellite peaks, which probably arise from the coordinated water molecules ( Supplementary Fig. 3b ). In contrast, the M2′ site consists of the side chains of Glu307 and Glu311, as well as the side chain of Asp348 and main chains of Arg345 and Asp346 in the symmetry-related molecule ( Fig. 2c ). The M3 site is located at the periplasmic entrance of the pore and is situated nearly on the twofold NCS axis. The Mn 2+ ion of this site is directly coordinated by the side-chain carboxylate group of Glu311 in one protomer and the main-chain carbonyl group of Glu311 of another protomer ( Supplementary Fig. 3e ). The M3 site is involved in crystal-packing interactions: the Mn 2+ ion is coordinated by the side-chain carboxylate group of Glu275 in the symmetry-related molecule ( Supplementary Fig. 3e ). In the crystal structure of the Ca 2+ -bound form, we observed a strong density peak only in the M3 site (2.9 σ, Supplementary Fig. 2f ), which may arise from the Ca 2+ ion. The Ca 2+ ion is directly coordinated by the side-chain carboxylate groups of Glu275 in the symmetry-related molecule and Glu311 ( Supplementary Fig. 3f ); however, the coordination manner is slightly different from that in the Mn 2+ -bound form ( Supplementary Fig. 3e ). By contrast, no strong density peaks were observed in the M2, M2′ and M3 sites in the Mg 2+ -bound structure ( Supplementary Fig. 3a,d ). Therefore, these observations suggested that these periplasmic cation-binding sites can discriminate divalent cations by directly coordinating them: the M3 site can bind both Mn 2+ and Ca 2+ , while the M2 (and M2′) site can bind Mn 2+ , but not Ca 2+ . Mg 2+ transport activity of MgtE and its mutants To investigate the role of the metal-binding sites in the TM domain, we analysed the ion-transport activity of wild-type (WT) MgtE and its mutants in vitro . We quantified the amounts of divalent cations accumulated within proteoliposomes reconstituted with MgtE or MgtE mutants, using the divalent cation-specific fluorescent indicator KMG-20. Although KMG-20 was developed as a Mg 2+ indicator [24] , it is also useful for the quantification of Ca 2+ and Mn 2+ ( Supplementary Fig. 4a,b ). At first, we measured the Mg 2+ transport activity of WT MgtE and the M1 site mutants (D432A and D432N). The results showed that the D432A and D432N mutants have no activity, as compared with the WT MgtE ( Fig. 3a ), consistent with the previous patch-clamp analysis results [16] . Next, we measured the activity of the M2 and M3 site mutants. In the M2A and M3A mutants, the residues involved in the cation binding (that is, Gln304, Glu307 and His383 for M2 and Glu311 for M3) are replaced by Ala, while all of these residues are replaced by Ala in the M2M3A mutant. The results showed that all of the M2A, M3A and M2M3A mutants possess comparable Mg 2+ transport activity to that of WT MgtE, suggesting that the M2 and M3 sites do not affect the Mg 2+ transport mechanism ( Fig. 3b and Supplementary Fig. 5 ). This is consistent with the crystal structure, in which Mg 2+ binding was disrupted at the M2 and M3 sites ( Supplementary Fig. 3a,d ). Therefore, these results indicated that the M1 site, but not the M2 and M3 sites, is directly involved in the Mg 2+ transport mechanism. 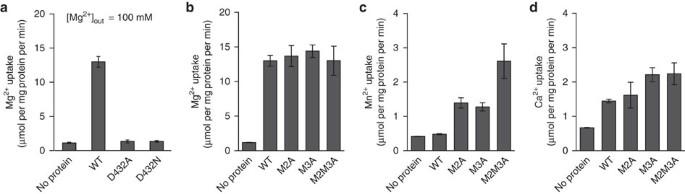Figure 3: Functional assays of MgtE reconstituted into liposomes. (a) Mg2+uptake by WT MgtE and its mutants in the presence of 100 mM MgCl2. (b–d) Divalent cation uptake by WT MgtE and its mutants in the presence of 100 mM Mg2+(b), Mn2+(c) and Ca2+(d). All data points are mean±s.e.m. (n=3). Figure 3: Functional assays of MgtE reconstituted into liposomes. ( a ) Mg 2+ uptake by WT MgtE and its mutants in the presence of 100 mM MgCl 2 . ( b – d ) Divalent cation uptake by WT MgtE and its mutants in the presence of 100 mM Mg 2+ ( b ), Mn 2+ ( c ) and Ca 2+ ( d ). All data points are mean±s.e.m. ( n =3). Full size image Cation selectivity of MgtE and its mutants To explore the ion selectivity of MgtE, we examined its Mn 2+ and Ca 2+ transport activities, using the liposome-based assay. WT MgtE exhibited almost no Mn 2+ transport activity, whereas the M2A and M3A mutants exhibited a 3.2-fold increase in Mn 2+ permeability, as compared with that of WT MgtE ( Fig. 3c ). The M2M3A mutant exhibited as much as a 5.2-fold increase over that of the WT MgtE ( Fig. 3c ). However, it should be noted that the Mn 2+ transport activity of the M2M3A mutant is still ~20% of that of Mg 2+ ( Fig. 3b,c ). The M2 and M3 sites may partly contribute to the low Mn 2+ transport by MgtE, and thus their disruption resulted in the increased permeability for Mn 2+ . It should be noted here that the disruption of the M3 site affected the Mn 2+ transport activity ( Fig. 3c ). This suggested that the M3 site also interacts with Mn 2+ in the lipid bilayer environment, although the Mn 2+ ion in the M3 site is coordinated by the Asp275 side chain in the symmetry-related molecule in the crystal ( Fig. 2c ). As for the Ca 2+ ion, the M3A and M2M3A mutants showed ~1.3-fold higher Ca 2+ transport activity than those of the WT and the M2A mutant ( Fig. 3d ). These results suggested that the M3 site, but not the M2 site, has a slight effect on the Ca 2+ transport activity. This is consistent with the observation in the crystal structure, in which Ca 2+ is bound to the M3 site ( Supplementary Fig. 3h ). Furthermore, we showed that both the WT and M2A mutant have almost no transport activity for Na + and K + , using Sodium Green and PBFI, respectively ( Supplementary Fig. 6a,b ). These results indicated that the M1 site strictly discriminates the monovalent and divalent cations. Taken together, the M1 site is mainly involved in the higher permeability of Mg 2+ over Mn 2+ and Ca 2+ by MgtE, which is further enhanced by the periplasmic cation-binding sites. Competitive inhibition of Mg 2+ transport activity by cations Next, to investigate the ion-selectivity mechanism by the M2 and M3 sites, we further examined the effects of Mn 2+ , Ca 2+ , Na + and K + on the Mg 2+ transport activity. The results revealed that Mn 2+ has a strong inhibitory effect on the transport activity of WT MgtE: the Mg 2+ transport activity decreased to ~33% in the presence of 1 μM Mn 2+ ( Fig. 4a ). A similar result was obtained with a fluorescent microscopy-based method, using MgtE-expressing giant spheroplasts ( Supplementary Fig. 7 ). This inhibitory effect is reduced in the M2A, M3A and M2M3A mutants, while a weak inhibitory effect still remains in the M2M3A mutant ( Fig. 4a ). These results suggested that the binding of Mn 2+ to the M2 and M3 sites strongly inhibits the Mg 2+ transport activity of MgtE. 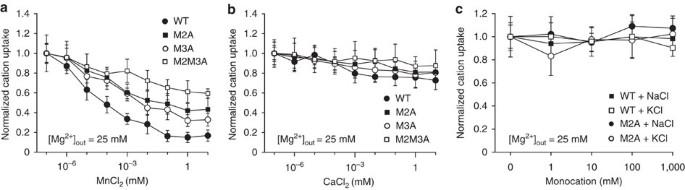Figure 4: Competition assay with Mn2+, Ca2+, Na+and K+. (a,b) Inhibition of the transport activity of WT MgtE and its mutants in the presence of 25 mM MgCl2and the indicated concentrations of Mn2+(a) and Ca2+(b). (c) Competition assay with Na+and K+of WT MgtE and the M2A mutant in the presence of 25 mM MgCl2and the indicated concentrations of monocations. All data points are mean±s.e.m. (n=3). Figure 4: Competition assay with Mn 2+ , Ca 2+ , Na + and K + . ( a , b ) Inhibition of the transport activity of WT MgtE and its mutants in the presence of 25 mM MgCl 2 and the indicated concentrations of Mn 2+ ( a ) and Ca 2+ ( b ). ( c ) Competition assay with Na + and K + of WT MgtE and the M2A mutant in the presence of 25 mM MgCl 2 and the indicated concentrations of monocations. All data points are mean±s.e.m. ( n =3). Full size image In contrast, Ca 2+ has only a small effect on the Mg 2+ transport activity of WT MgtE, as compared with Mn 2+ ( Fig. 4b ). Moreover, similar results were obtained with all of the M2A, M3A and M2M3A mutants. Thus, these results suggested that the presence of Ca 2+ has almost no inhibitory effect on the Mg 2+ transport activity, and that Ca 2+ binding to the M3 sites does not inhibit the Mg 2+ transport activity. In the competition assay using Na + and K + , the Mg 2+ transport activity was not affected by Na + and K + , even at concentrations over 1 M ( Fig. 4c ). These monovalent cations may have much lower affinity than Mg 2+ to the M1 site, and thus are not transported by MgtE. These observations indicated that the periplasmic cation-binding sites are mainly involved in the selectivity of divalent cations. Gating mechanism by the periplasmic cation-binding site Given that the periplasmic cation-binding sites are formed across the dimer interface ( Fig. 2c ), the binding of divalent cations can fix the arrangement of the MgtE protomers in the closed form, which may prevent the ion conduction. To assess this hypothesis, we performed the single-channel analysis using the patch-clamp technique. The results showed that the presence of Mn 2+ on the periplasmic side significantly decreases the open-channel probability of the WT MgtE channel, while such a change in the open-channel probability was not observed in the M2A mutant ( Fig. 5 ). Thus, the low permeability of MgtE in the presence of Mn 2+ ( Fig. 4a ) is mainly ascribed to the change in the open probability of the channel. The Mn 2+ binding to the M2 site may stabilize the closed form of MgtE, thereby preventing the opening of the cation-conducting pore. 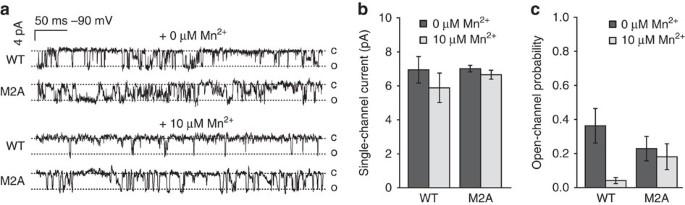Figure 5: Single-channel analysis of WT MgtE and the M2A mutant by the patch-clamp technique. (a) Current traces of WT MgtE and the M2A mutant in the inside-out configuration at –90 mV, in the presence and absence of 10 μM Mn2+on the periplasmic side. C and O indicate the closed and open states of MgtE, respectively. (b,c) Single-channel current (b) and open-channel probability (c) of WT MgtE and the M2A mutant in the presence and absence of 10 μM Mn2+on the periplasmic side. Figure 5: Single-channel analysis of WT MgtE and the M2A mutant by the patch-clamp technique. ( a ) Current traces of WT MgtE and the M2A mutant in the inside-out configuration at –90 mV, in the presence and absence of 10 μM Mn 2+ on the periplasmic side. C and O indicate the closed and open states of MgtE, respectively. ( b , c ) Single-channel current ( b ) and open-channel probability ( c ) of WT MgtE and the M2A mutant in the presence and absence of 10 μM Mn 2+ on the periplasmic side. Full size image Periplasmic cation-binding sites of MgtEs from other species The MgtEs from several species also have acidic and/or hydrophilic residues around the M2 and M3 sites, as suggested from the amino-acid sequence alignment and the homology modelling ( Supplementary Figs 2 and 8a ). Thus, it is likely to be that the acidic and/or hydrophilic residues of these MgtEs also form cation-binding sites and thereby function as periplasmic gating sites. To test this hypothesis, we analysed the Mg 2+ and Mn 2+ transport activities of the WT MgtE and its mutants (M2A and M3A mutants) from Methanosarcina mazei (MmMgtE), which seems to have structurally conserved M2 and M3 sites ( Supplementary Figs 2 and 8a ). In the M2A and M3A mutants, the acidic and/or hydrophilic residues around the M2 and M3 sites (that is, Glu300 and Glu378 for M2 and Gln304 for M3) are replaced by Ala, while all of these residues are replaced by Ala in the M2M3A mutant. The results showed that the WT MmMgtE has similar Mg 2+ transport activity as that of T. thermophilus MgtE (TtMgtE), while it has almost no Mn 2+ transport activity ( Supplementary Fig. 8b,c ). Furthermore, the M2A and M3A mutants of MmMgtE showed about two- and threefold higher Mn 2+ transport activities than that of the WT, respectively, as observed in the case of TtMgtE ( Supplementary Fig. 8b,c ). Thus, these results support our proposal that the M2 and M3 sites of MmMgtE also function as periplasmic gating sites. Next, to further verify our hypothesis, we analysed the effects of Mn 2+ on the Mg 2+ transport activity of MmMgtE and its mutants. The results showed that the Mg 2+ transport activity of the WT MmMgtE decreased to ~42% in the presence of 1 μM Mn 2+ ( Supplementary Fig. 8d ), and this inhibitory effect was reduced in the M2A and M3A mutants ( Supplementary Fig. 8d ). Therefore, these observations strongly support our proposal that Mn 2+ binding to the M2 and M3 sites inhibits the Mg 2+ transport activity of MmMgtE, as observed in the case of TtMgtE. Taken together, the M2 and M3 sites are structurally and functionally conserved among the MgtEs, while they are not strictly conserved at the amino-acid sequence level. In this work, we determined the high-resolution crystal structures of MgtE-TMD bound to Mg 2+ , Mn 2+ and Ca 2+ , and performed biochemical analyses based on the structures. The crystal structure of the Mg 2+ -bound form revealed that the M1 site recognizes the Mg 2+ ion in a fully hydrated state. The structure suggested that the M1 site, including the carboxylate groups of the Asp432 side chains, strictly recognizes the size and geometry of the Mg 2+ hydration shells, which may be important for the selective transport of Mg 2+ over other cations, such as Na + , K + and Ca 2+ . The present crystal structure of MgtE-TMD is essentially the same as that of the full-length MgtE in the closed conformation. The hydrophobic gate located just above the M1 site is closed in the structure of MgtE-TMD, whereas the M1 site is accessible from the cytosolic side ( Fig. 1b ). Thus, in the open-form of MgtE, this hydrophobic gate will be open to permeate ions and Asp432 will become accessible from the extracellular side. Our previous patch-clamp analysis results demonstrated the high Mg 2+ conductivity of MgtE (96 pS), which is similar to that of the prokaryotic potassium channel KcsA (20~100 pS) [16] , [25] , [26] . Therefore, the opening of the hydrophobic gate may be large enough to accommodate the fully hydrated Mg 2+ ion. Here we hypothesized that the structure of the selectivity filter (that is, the M1 site) in the present structure is also conserved in this open-form MgtE, as in the cases of other channels, including KcsA [27] ( Fig. 6a ). Based on this hypothesis, the present crystal structure excellently explains the cation selectivities of the M1 site of MgtE for the biological cations, Na + , K + , Mg 2+ and Ca 2+ , observed in the present biochemical analysis using the M2M3A mutant. The size of the fully hydrated Mg 2+ ion (~6 Å) is slightly larger than the constriction between the Asp432 residues (~5 Å) in the MgtE pore. The electrostatic interaction between Mg 2+ and the −2 charge of Asp432 in the M1 site is strong enough to decrease the steric barrier of this constriction, thereby enabling the high Mg 2+ conductivity. The hydrogen bonds between the M1 site and the water molecules in the first- and second-hydration shells may further reduce this steric barrier ( Fig. 6a ). In contrast, the radius of the first hydration shell of the Ca 2+ ion is larger than that of Mg 2+ , which may prevent its efficient transport. In addition, the formation of specific hydrogen bonds between the M1 site and the water molecules coordinated to Ca 2+ is geometrically impossible, which may also increase the barrier for Ca 2+ to pass through the M1 site. Furthermore, in the case of the monovalent cations, the electrostatic interaction between the monovalent cations and the –2 charge of Asp432 in the M1 site is weaker than that of the divalent cations, which may prevent the interaction of the monovalent cations with the M1 site. 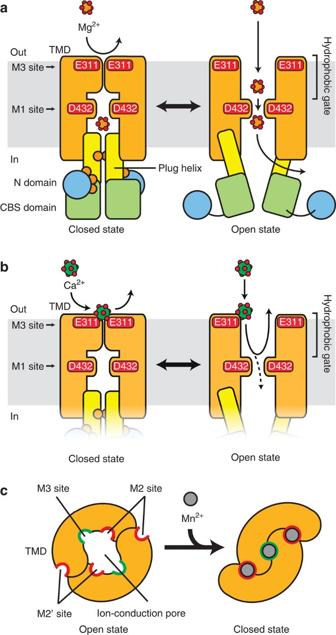Figure 6: Proposed model for the ion-conduction mechanism of MgtE. (a) Model for the Mg2+transport mechanism. A schematic representation of MgtE, viewed from the plane in the membrane, is shown. The Mg2+binding to the cytosolic domain stabilizes the MgtE in the closed state (left panel), while the M2 and M3 sites do not bind to Mg2+, and thus the periplasmic Mg2+does not affect the gating of MgtE. After the dissociation of Mg2+from the cytosolic domain, MgtE adopts the open form (right panel). In the open form, the electrostatic interaction between Asp432 and Mg2+, and the hydrogen bonds between Asp432 and the Mg2+hydration shells enable the precise recognition and high-speed conduction of Mg2+. (b) Model for the Ca2+conduction mechanism. Solid and dashed lines represent the major and minor ion pathways for Ca2+, respectively. Although periplasmic Ca2+can interact with the M3 site, its weak affinity does not stabilize MgtE in the closed form (left panel). In the open form (right panel), Ca2+cannot pass through the selectivity filter (that is, Asp432) efficiently, because the interaction between Asp432 and its hydration shell is not optimal. The interaction between the M3 site and Ca2+also contributes to the slowing of its transport rate. The major portion of Ca2+diffuses back to the periplasmic side through the hydrophobic gate, while a small portion overcomes the barrier in the selectivity filter, which results in the weak Ca2+transport activity of MgtE. (c) Gating model of the ion-conducting pore by the periplasmic gating sites. A schematic representation of MgtE, viewed from the periplasmic side, is shown. Periplasmic Mn2+binds to the M2, M2′ and M3 sites with high affinity, which fixes MgtE in the closed form. This results in the high selectivity for Mg2+over Mn2+. Figure 6: Proposed model for the ion-conduction mechanism of MgtE. ( a ) Model for the Mg 2+ transport mechanism. A schematic representation of MgtE, viewed from the plane in the membrane, is shown. The Mg 2+ binding to the cytosolic domain stabilizes the MgtE in the closed state (left panel), while the M2 and M3 sites do not bind to Mg 2+ , and thus the periplasmic Mg 2+ does not affect the gating of MgtE. After the dissociation of Mg 2+ from the cytosolic domain, MgtE adopts the open form (right panel). In the open form, the electrostatic interaction between Asp432 and Mg 2+ , and the hydrogen bonds between Asp432 and the Mg 2+ hydration shells enable the precise recognition and high-speed conduction of Mg 2+ . ( b ) Model for the Ca 2+ conduction mechanism. Solid and dashed lines represent the major and minor ion pathways for Ca 2+ , respectively. Although periplasmic Ca 2+ can interact with the M3 site, its weak affinity does not stabilize MgtE in the closed form (left panel). In the open form (right panel), Ca 2+ cannot pass through the selectivity filter (that is, Asp432) efficiently, because the interaction between Asp432 and its hydration shell is not optimal. The interaction between the M3 site and Ca 2+ also contributes to the slowing of its transport rate. The major portion of Ca 2+ diffuses back to the periplasmic side through the hydrophobic gate, while a small portion overcomes the barrier in the selectivity filter, which results in the weak Ca 2+ transport activity of MgtE. ( c ) Gating model of the ion-conducting pore by the periplasmic gating sites. A schematic representation of MgtE, viewed from the periplasmic side, is shown. Periplasmic Mn 2+ binds to the M2, M2′ and M3 sites with high affinity, which fixes MgtE in the closed form. This results in the high selectivity for Mg 2+ over Mn 2+ . Full size image The present results also suggested that the M3 site is involved in the low Ca 2+ permeability: the M3A mutant exhibited higher Ca 2+ transport activity than that of the WT MgtE ( Fig. 3d ). However, in the competition assay, Ca 2+ had almost no inhibitory effect on the Mg 2+ transport activities of both the WT MgtE and its mutants ( Fig. 4b ). This result suggested that unlike Mn 2+ , Ca 2+ does not strongly bind to the TM pore of MgtE to fix the conformation of MgtE in the closed state ( Fig. 6b ). The M3 site may contribute to the low Ca 2+ permeability, transiently trapping Ca 2+ at the entrance of the cation-conducting pore of MgtE ( Fig. 6b ). Numerous crystal structures of ion channels have revealed the structural bases for their ion selectivity mechanisms. Particularly, the atomic-resolution crystal structures and functional analyses of the voltage-gated K + channel superfamily, including KcsA [3] , [4] , MthK [5] and NaK [28] , provided insights into the ion selectivity mechanism of K + : the backbone carbonyl oxygen atoms recognize the cations in the dehydrated forms. In striking contrast, the present crystal structure revealed that the fully hydrated Mg 2+ ion is recognized by the Asp432 side chains in the M1 site of MgtE, which is quite different from the cases of the monovalent cations. The proper arrangement of the two carboxylate groups in the M1 site may strictly recognize the specific hydration-shell structure of the Mg 2+ ion, thereby enabling the selective transport of Mg 2+ over other biological cations. This MgtE mechanism seems to be reasonable for the fast and selective conduction of Mg 2+ , as the energy required for the dehydration of divalent cations is four to five times higher than that of monovalent cations [29] . Moreover, it was proposed that Mg 2+ channel CorA also transport Mg 2+ ion in a fully hydrated form, based on its inhibition by the Co 2+ hexammin compound [8] . Thus, selectivity based on the hydrated Mg 2+ may be a common feature of Mg 2+ channels. Transition metal cations, such as Fe 2+ , Co 2+ , Ni 2+ and Mn 2+ , are important as essential trace elements, but overexposure to them is toxic for living organisms. The present crystal structure revealed that Mn 2+ bound to the M2 and M3 sites. The direct interaction between the cation and the protein ligand atoms, including the carbonyl oxygens of Glu307 and Gln304, and the imidazole nitrogen atoms of His383, may enable the discrimination between Mn 2+ and Mg 2+ . The functional analysis revealed that Mn 2+ binding to the M2 and M3 sites strongly inhibits the cation transport activity of MgtE. The patch-clamp analysis further showed that the presence of Mn 2+ on the periplasmic side decreases the open probability of the channel ( Fig. 5 ). Therefore, the binding of transient-metal cations, including Mn 2+ , to these periplasmic gating sites (that is, M2 and M3 sites) may fix the arrangement of the MgtE protomers in the closed form, thereby preventing the excess uptake of these toxic cations ( Fig. 6c ). The present work further suggested the presence of these periplasmic gating sites in MgtEs from other species, including M. mazei ( Supplementary Fig. 8 ). In addition, we found that the M2M3A mutant, which disrupts all of the periplasmic gating sites, still preferably transports Mg 2+ over Mn 2+ ( Fig. 3b,c ). The results of the competitive inhibition analysis further showed that Mn 2+ has an inhibitory effect on the cation transport activity of the M2M3A mutant ( Fig. 4a ). These results suggested that the M1 site has higher affinity for Mn 2+ than Mg 2+ . The higher affinity may trap Mn 2+ in the M1 site, which may result in the decreased Mg 2+ permeability in the presence of Mn 2+ , as well as the Mn 2+ conductance itself. However, it seems to be difficult to explain this difference in the affinity from only the present crystal structure: both Mg 2+ and Mn 2+ bind to the M1 site in similar manners, in which the Asp432 carboxylate groups indirectly recognize these cations through the water molecules in their first hydration shell ( Figs 1c and 2a ). Thus, the question arises as to what causes this difference in the affinity of the M1 site for the fully hydrated Mg 2+ and Mn 2+ ions. Previous quantum chemical calculations of Mg 2+ and Mn 2+ in complex with water molecules revealed that the hydration geometry of the Mn 2+ ion deviates from the ideal octahedral arrangement, due to the excessive polarization and charge-transfer effects of Mn 2+ with open d orbitals [30] , [31] . This difference between Mg 2+ and Mn 2+ was suggested to affect the substrate specificity of restriction enzymes [32] . We expect that this difference in the electronic states and polarization would also contribute to the difference in the affinities of the M1 site for Mg 2+ and Mn 2+ . Further understanding of the discrimination mechanism of Mg 2+ and transition metal cations will require structural and computational analyses, including ab initio quantum chemical calculations. Overall, our study provides structural insights into the specific recognition of Mg 2+ over other cations by the MgtE Mg 2+ channel, to achieve fast and selective ion permeation in combination with the selectivity filter, M1, and the periplasmic gating sites, M2 and M3. Expression and purification Full-length T. thermophilus MgtE (TtMgtE) was subcloned into a pET-modified vector, including an amino-terminal His 6 tag [16] , [17] . The tobacco etch virus (TEV) protease cleavage site was inserted into the L0 loop, which connects the cytosolic and TM domains of TtMgtE, by PCR with the primers 5′-ATTTTCAAGGAGTGCCCGACCTCGTCTACAGCGAGG-3′ and 5′-TATTTAAAAGCAGGTGCCGCGGCTCGAACACCTAC-3′. The protein was overexpressed in Escherichia coli C41 (DE3) cells, induced with 0.5 mM isopropyl D -thiogalactoside for 18 h at 20 °C. The cells were disrupted and the membrane fraction was collected by ultracentrifugation. This fraction was solubilized by 1.5% (w/v) n-dodecyl-beta-D-maltopyranoside (DDM) in buffer A (50 mM HEPES (pH 7.0), 300 mM NaCl and 20 mM imidazole). The solubilized fraction was applied to a Ni-NTA column equilibrated with buffer A containing 0.1% (w/v) DDM and mixed for 30 min. The column was washed with buffer A containing 0.1% (w/v) DDM and 50 mM imidazole, and TtMgtE was eluted in the same buffer containing 250 mM imidazole. To cleave the TEV protease cleavage site, the purified MgtE was treated with His 6 -tagged TEV protease and dialysed against buffer B (25 mM HEPES (pH 7.0), 150 mM NaCl, 0.1% (w/v) DDM). The sample was reloaded on a Ni-NTA column equilibrated with buffer B, to remove the cytosolic domain and the TEV protease. The flow-through fraction containing the TM domain of MgtE (MgtE-TMD) was collected and further purified by chromatography on a Superdex200 10/300 column in buffer B. The purified MgtE-TMD was concentrated to ~10 mg ml −1 , using an Amicon Ultra 50K filter. Crystallization For the lipidic cubic phase (LCP) crystallization trials [19] , we used monoolein (Sigma) or 7.7MAG [33] as the host lipid. MgtE-TMD was mixed with the host lipid in a 2:3 protein to lipid ratio (w/w), using the twin-syringe mixing method. Aliquots (100 nl) of the protein–LCP mixture were spotted on a 96-well sandwich plate and overlaid by 800 nl of precipitation solution by the crystallization robot, mosquito LCP (TTP LabTech). Crystals for data collection were grown at 20 °C in monoolein, with a reservoir containing 30–35% (w/v) PEG600, 100 mM Tris (pH 8.0), 120 mM Mg-formate and 100 mM NaCl. For crystallization in the presence of Mn 2+ and Ca 2+ , the purified protein solution was diluted to a DDM concentration of 0.05% and was concentrated to ~10 mg ml –1 . Crystals were obtained as described above, in a reservoir containing 30–32% (w/v) PEG300, 100 mM HEPES-NaOH (pH 7.5) and 80–120 mM MnCl 2 , and a reservoir containing 20–28% (w/v) PEG400, 100 mM HEPES (pH 7.5), 120–160 mM CaCl 2 and 100 mM NaSCN. Data collection and structure determination All diffraction data sets were collected at the SPring-8 BL32XU (Hyogo, Japan). The data sets were processed with the programmes HKL2000 (HKL Research, Inc.) and XDS [34] . Phases were obtained by molecular replacement with the programme MOLREP [35] , using the TM domain of the previous MgtE coordinates (PDB 2ZY9) as a search model. The model was subsequently improved through iterative cycles of manual building with COOT and refinement with the programme PHENIX [36] . The structural refinement statistics are summarized in Table 1 . Molecular graphics were illustrated with CueMol ( http://www.cuemol.org/ ). Divalent cation uptake assay The divalent cation uptake assay was performed as previously described [37] , with some modifications. Purified WT and mutant TtMgtE proteins were reconstituted into liposomes at a 50:1 E. coli polar lipid to protein ratio (w/w), by the freeze–thaw method. The proteoliposomes were loaded with buffer C (25 mM HEPES (pH 7.0), 100 mM NaCl) and the reaction was initiated by adding MgCl 2 . After an incubation for 20 min at room temperature, 2 mM Co(III)hexamine was added to stop the cation uptake through the MgtE protein [16] . The reaction mixture was centrifuged at 210,000 g for 10 min. The pellet was washed three times in buffer C containing 2 mM Co(III)hexamine and was resuspended in buffer C containing 0.5% SDS. The suspension was mixed with 10 μM divalent cation indicator, KMG-20 (ref. 24 ) (Wako), and incubated for 2 h at 37 °C. The KMG-20 fluorescence was excited at 440 nm and detected at 500–530 nm, using an F-7000 fluorescence spectrophotometer (Hitachi). Divalent cation uptake was calculated from a Benesi–Hildebrand plot [24] , obtained from the known concentration of each indicated divalent cation in buffer C containing 0.5% SDS. NaCl and KCl have no effect on the fluorescence intensity of KMG-20 (ref. 24 ). In the previous report [16] , divalent cation binding to the cytosolic domain strongly stabilized the closed state of the ion-conducting pore at concentrations over 10 mM. Thus, in this experiment, the MgtE with the cytosolic domain facing towards the extraliposomal side does not contribute to the Mg 2+ transport activity, because we measured the activity under conditions with an extraliposomal Mg 2+ concentration higher than 10 mM. Na + and K + uptake assays The Na + and K + uptake assays were performed as previously described [38] , [39] , [40] . Briefly, E. coli polar lipids and ergosterol, at a 50:1 ratio (w/w), were suspended in buffer D (25 mM Tris (pH 7.5), 100 mM n-methyl-D-glucamin) with 10 μM Sodium Green and 60 μM PBFI, respectively, and sonicated with a large tip for 30 s. The liposome solution was centrifuged at 210,000 g for 10 min and the pellet was resuspended in buffer D. The purified WT MgtE, the M2A mutant and the Na + ionophore, a nystatin–ergosterol complex (10 nmol) [41] , were reconstituted into liposomes by the freeze–thaw method. The liposomes were centrifuged at 210,000 g for 10 min and the pellet was resuspended in buffer D. The Na + and K + uptake reactions were initiated by the addition of NaCl and KCl, respectively, and were monitored by the fluorescence of Sodium Green ( λ ex / λ em =488/540) and PBFI ( λ ex / λ em =493/515), respectively. Patch-clamp analysis E. coli giant spheroplasts were prepared as described previously [16] . Spheroplasts expressing WT MgtE and the M2A mutant were plated on glass coverslips in a bath medium (250 mM N-methyl- D -glucamine, 40 mM MgCl 2 , 300 mM glucose and 10 mM HEPES, pH 7.2). Borosilicate pipettes (Harvard Apparatus, Kent, UK), with about 5–8 MΩ resistance, were filled with a pipette solution (250 mM N-methyl- D -glucamine, 40 mM MgCl 2 , 300 mM glucose and 10 mM HEPES, pH 7.2). In some experiments, 10 μM MnCl 2 was added to the pipette solution. After the formation of a gigaseal, a membrane patch was excised and the bath solution was exchanged using a perfusion system with a batch solution: 250 mM N-methyl- D -glucamine, 0.2 mM MgCl 2 , 300 mM glucose and 10 mM HEPES, pH 7.2. The membrane patch voltage was clamped and currents were recorded using an Axopatch 200B amplifier (Axon CNS, Molecular Devices), coupled to an A/D converter (Axon CNS, Molecular Devices) and controlled by the pclamp10 software (Axon CNS, Molecular Devices). Currents were filtered at 2 kHz and sampled at 5 kHz. Time-lapse analysis of magnesium fluorescence Spheroplasts were loaded with 2 μM Mag-Fluo4-AM (Life Technologies, USA) for 45 min. The spheroplasts were then centrifuged at 4,000 r.p.m. to remove the excess Mag-Fluo4 and resuspended in a buffer containing 150 mM KCl, 10 mM HEPES and 300 mM sucrose, pH 7.4. The spheroplasts were then placed on a glass coverslip under an inverted microscope with a × 60 water immersion objective (Olympus IX71, Olympus, Japan). For the time-lapse monitoring of Mag-Fluo4 fluorescence, the probe was excited with 488 nm illumination generated by a monochromator (Polychrome V, TILL Photonics, Germany). The camera and monochromator were controlled with the Metafluor imaging software (Molecular Devices, USA). Mag-Fluo4 fluorescent emissions at 535 nm were then collected with an Orca Flash 2.8 CMOS camera (Hamamatsu, Japan) every 2 s and this experiment was repeated five times. Accession codes: Atomic coordinates and structure factors for the T. ther MgtE bound to Mg 2+ , Mn 2+ and Ca 2+ have been deposited in the Protein Data Bank, under the accession codes 4U9L, 4U9N and 4WIB, respectively. How to cite this article: Takeda, H. et al. Structural basis for ion selectivity revealed by high-resolution crystal structure of Mg 2+ channel MgtE. Nat. Commun. 5:5374 doi: 10.1038/ncomms6374 (2014).